Dynamic strain-mediated coupling of a single diamond spin to a mechanical resonator The development of hybrid quantum systems is central to the advancement of emerging quantum technologies, including quantum information science and quantum-assisted sensing. The recent demonstration of high-quality single-crystal diamond resonators has led to significant interest in a hybrid system consisting of nitrogen–vacancy centre spins that interact with the resonant phonon modes of a macroscopic mechanical resonator through crystal strain. However, the nitrogen–vacancy spin–strain interaction has not been well characterized. Here, we demonstrate dynamic, strain-mediated coupling of the mechanical motion of a diamond cantilever to the spin of an embedded nitrogen–vacancy centre. Via quantum control of the spin, we quantitatively characterize the axial and transverse strain sensitivities of the nitrogen–vacancy ground-state spin. The nitrogen–vacancy centre is an atomic scale sensor and we demonstrate spin-based strain imaging with a strain sensitivity of 3 × 10 −6 strain Hz −1/2 . Finally, we show how this spin-resonator system could enable coherent spin–phonon interactions in the quantum regime. Nitrogen–vacancy (NV) centres in diamond are among the most promising implementations of quantum bits for quantum information processing [1] and nanoscale field sensors [2] . Because of their excellent coherence properties [3] and their ability to coherently couple to various external fields, NV centres are ideal candidates for integration into a hybrid quantum system, which combines the merits of two or more physical systems to mitigate their individual weaknesses. To date, experimental efforts have focused on integrating the NV centre into hybrid systems consisting of photons [4] , [5] , [6] , nuclear spins [7] and magnetically coupled mechanical resonators [8] , [9] . Recent demonstrations of high-quality ( Q ) factor single-crystal diamond (SCD) mechanical resonators [10] , [11] have generated interest in the development of a monolithic structure consisting of such a resonator that is strain coupled to the electronic spin of an embedded NV centre [12] , [13] . With the NV’s long quantum coherence time and diamond’s low-mechanical losses, this system provides a unique environment to engineer spin–spin entanglement or spin squeezing [12] . Moreover, a coherent spin–phonon interaction may be used to generate non-classical states of the resonator, such as Schrödinger cat states [13] , [14] , [15] , [16] . An inherent advantage of a strain-coupled spin-resonator system is the intrinsic nature of the coupling; no additional components are required to tune the coupling strength, such as an atomic force microscope tip or cavity, which may introduce fluctuating fields that decohere the NV spin. In addition, in contrast with other hybrid mechanical systems, this NV-resonator system requires no functionalization of the resonator with, for example, a mirror or electrode, which could adversely affect the Q . However, to engineer such a system, we require a quantitative understanding of how strain couples to the ground-state spin levels of the NV centre. Despite the NV’s well-understood sensitivity to magnetic [2] and electric [17] , [18] fields and temperature [19] , [20] , the NV ground-state strain sensitivity has not been fully characterized, and there exist competing theoretical models of the strain interaction [18] , [21] , [22] , [23] . In this letter, we use high- Q SCD cantilevers to probe the interaction between a single NV spin and crystal strain. The magnitude of the strain is highly controlled, and is set by the cantilever’s mode shape and amplitude of motion, the depth and lateral location of the NV in the cantilever and the orientation of the NV with respect to the cantilever axis. The strain induced by an oscillating cantilever modulates the energy of the ground-state spin levels, which is detected via coherent quantum control of the spin [24] . Combined with the known strain profile of a cantilever under pure bending and the four possible NV orientations in the diamond crystal structure, our measurements allow us to extract the axial and transverse strain susceptibilities. Thus, the NV is a calibrated strain sensor, with which we image the strain profile of the resonator. Importantly, we demonstrate NV–strain coupling in a geometry appropriate for realizing a hybrid quantum system, and show that by scaling down the dimensions of the resonator, it should be possible to reach the quantum regime of coupling between spins and phonons. Strain model and experimental setup Here, we model strain by an effective electric field in which strain-induced displacements of the atoms alter the electron density in the crystal, resulting in local electric fields [17] , [18] . Therefore, the ground-state Hamiltonian for an NV in the presence of magnetic and strain fields may be described by ( h =1) where D 0 is the crystal-field splitting ( D 0 =2.87 GHz), γ NV is the gyromagnetic ratio ( γ NV =2.8 MHz G −1 ), d ‖ and d ⊥ are the strain susceptibility parameters parallel and perpendicular to the NV symmetry axis (whose values are determined in this work), S ± are the spin-1 raising and lowering operators, , , and are the diagonal components of the strain tensor defined in the NV’s basis (note we have neglected shear). We will henceforth refer to d ‖ and d ⊥ as the axial and transverse strain susceptibility parameters. A uniaxial strain along the NV symmetry axis, results in a shift of the crystal-field splitting, whereas a strain transverse to the symmetry axis, results in mixing between the eigenstates. Because strain and stress are tensors, the uniaxial stress due to the bending of the cantilever will generate strain along all three principal directions because of the Poisson effect [25] . This effect cannot be neglected, as shown later. In this experiment, an NV interacts with the fundamental mechanical mode of the cantilever via strain ( Fig. 1a ). For small displacements of the cantilever, the strain felt by the NV centre is linear in cantilever position, and the total strain can be written as , where X d is the amplitude of driven motion, x 0 is the amplitude of zero point motion and is the strain induced by the zero point motion [12] . 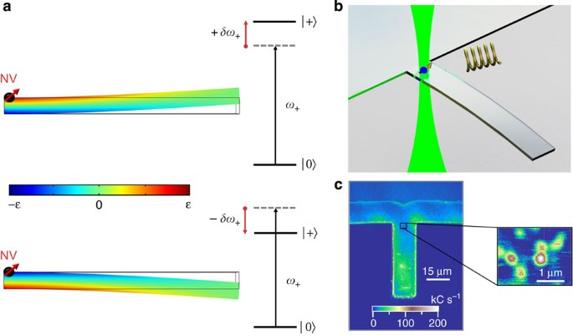Figure 1: A hybrid NV-cantilever system. (a) Strain modulates the spin levels of an NV centre embedded in a cantilever. The strain profile was simulated using a finite element method. (b) Schematic of experiment: a green laser is focused onto a single NV spin embedded in a cantilever via a confocal microscope for initialization and readout. Microwaves are used for pulsed spin manipulation. (c) Confocal image of a cantilever showing the presence of single embedded NV centres. If the NV is in the presence of a static magnetic field aligned closely to its symmetry axis, equation (1) can be approximately diagonalized with eigenstates , and the energies can be expressed as a function of the normalized beam displacement, Figure 1: A hybrid NV-cantilever system. ( a ) Strain modulates the spin levels of an NV centre embedded in a cantilever. The strain profile was simulated using a finite element method. ( b ) Schematic of experiment: a green laser is focused onto a single NV spin embedded in a cantilever via a confocal microscope for initialization and readout. Microwaves are used for pulsed spin manipulation. ( c ) Confocal image of a cantilever showing the presence of single embedded NV centres. Full size image where and are the axial and transverse strain couplings to the zero point motion of the resonator, and are defined as ( Supplementary Note 1 ), where α /2 is the Stückelberg angle and . We note that by tuning B z we may selectively characterize axial and transverse strain, as evidenced in equation (2). The experiment consists of a single spin embedded in a SCD cantilever ( Fig. 1b ). The cantilevers used here ( Fig. 1c ) were fabricated using the technique described in ref. 10 , and are 60 μm long, 15 μm wide and ~1 μm thick. They have fundamental frequencies ω m /2π near 1 MHz and quality factors exceeding 3.0 × 10 5 , which were measured using optical interferometry [10] . All measurements were performed at room temperature and at pressures of approximately 10 −5 Torr. NVs were formed approximately 50 nm below the diamond surface via 14 N ion implantation and vacuum annealing (see Methods). The orientation of the NV with respect to the cantilever ( Supplementary Fig. 1 ) is identified through its Zeeman splitting in an applied static magnetic field. We align this field closely to the NV axis to break the degeneracy of the spin levels. We encode our qubit in the and spin states, and coherently manipulate the spin using near-resonant microwaves. We are able to distinguish the effects of and by noting an AC ε ‖ modulates the qubit frequency at ω m , whereas an AC modulates the qubit frequency at approximately 2 ω m . 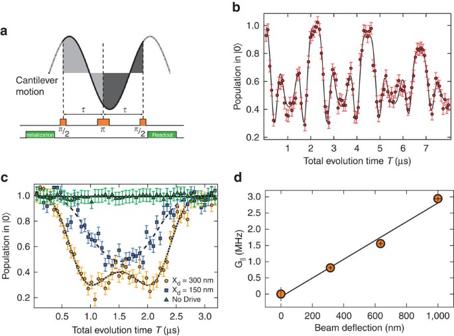Figure 2: Axial strain detection with a single NV. (a) AC axial strain is detected with a Hahn echo sequence. Transverse strain is suppressed by an applied 22 G axial magnetic field. The π pulse allows the phases from the first (light grey) and second (dark grey) free evolution periods to add constructively. (b) Measured Hahn echo spin population (red circles) for an NV at the base of a cantilever withand an oscillation amplitude of 650 nm as a function of total evolution timeT=2τ. The echo signal is given by a zero-order Bessel function (fit is black solid line) because the cantilever motion is not phase-locked to the timing of the control pulses. Error bars correspond to standard error in photon counting. (c) The amplitude of cantilever motion impacts the spin evolution. Hahn echo spin population of an NV at the base of acantilever in the absence of drive (green triangles), with a drive corresponding to 150 nm cantilever amplitude (blue squares) and 300 nm amplitude (yellow circles). Dotted black lines are fits to the data. (d) Plotted strain couplingG‖for an NV 11 μm from the base on the cantilever described inbas a function of beam deflection. Vertical error bars correspond to standard error of the fit to the theoretical echo signal. Horizontal error bars correspond to the uncertainty in beam deflection from interferometric measurements. Axial strain detection Figure 2a shows the measurement protocol for axial strain detection. The cantilever is resonantly driven with a piezoelectric transducer, and the phase of the drive is not phase-locked to the timing of the control pulses. The NV spin is initialized to the state via optical pumping with a 532 nm laser. Microwaves tuned to the transition are applied to the NV to carry out a Hahn echo pulse sequence with a total free evolution time T =2 τ . During the free evolution periods, the resonantly driven motion of the cantilever imprints a relative phase onto the qubit, which is then converted into a population difference and read out via the spin-dependent fluorescence. In the measurements of axial strain, B z was set to 22 G to suppress the effects of transverse strain, as shown in equation (2). Figure 2: Axial strain detection with a single NV. ( a ) AC axial strain is detected with a Hahn echo sequence. Transverse strain is suppressed by an applied 22 G axial magnetic field. The π pulse allows the phases from the first (light grey) and second (dark grey) free evolution periods to add constructively. ( b ) Measured Hahn echo spin population (red circles) for an NV at the base of a cantilever with and an oscillation amplitude of 650 nm as a function of total evolution time T =2 τ . The echo signal is given by a zero-order Bessel function (fit is black solid line) because the cantilever motion is not phase-locked to the timing of the control pulses. Error bars correspond to standard error in photon counting. ( c ) The amplitude of cantilever motion impacts the spin evolution. Hahn echo spin population of an NV at the base of a cantilever in the absence of drive (green triangles), with a drive corresponding to 150 nm cantilever amplitude (blue squares) and 300 nm amplitude (yellow circles). Dotted black lines are fits to the data. ( d ) Plotted strain coupling G ‖ for an NV 11 μm from the base on the cantilever described in b as a function of beam deflection. Vertical error bars correspond to standard error of the fit to the theoretical echo signal. Horizontal error bars correspond to the uncertainty in beam deflection from interferometric measurements. Full size image A dynamic axial strain results in a modulation of the spin population difference that is correlated to the motion of the cantilever. As depicted in Fig. 2b , when the total evolution time of the spin is equal to an odd integer multiple of the cantilever period, the accumulated phase is maximized, resulting in a reduced population in . When the total evolution time is equal to an even multiple of the cantilever period, the qubit acquires no phase, resulting in a revival of state population. Because the cantilever’s motion and microwave pulse timing are not phase locked, the signal averages over a uniformly distributed initial phase of the motion, and is given by a zero order Bessel function ( Supplementary Note 2 ). By fitting the data in Fig. 2b (solid black line) to the expected echo signal, we extract an axial strain coupling G ‖ = g ‖ X =2.1±0.1 MHz and a cantilever frequency , in agreement with the driving frequency of the cantilever of 884.583 kHz. The strain coupling can be tuned with cantilever drive. Figure 2c shows a Hahn echo measurement of a single NV for different beam deflection amplitudes. In the absence of cantilever drive, the spin retains its coherence over a single period of the cantilever’s motion. As the amplitude of driven motion increases, the increased strain coupling results in a reduced state population. For sufficiently high couplings, Bessel fringe oscillations are observed, indicating that the spin has precessed more than once around the equator of the Bloch sphere. In Fig. 2d , we plot G ‖ for four different drive amplitudes and confirm that the coupling is linear with beam displacement. Single spin strain imaging With its atom-sized spatial extent, the NV is a novel, nanoscale strain sensor. We demonstrate NV-based strain imaging by measuring G ‖ for several NVs located at different positions along the length of the cantilever ( Supplementary Fig. 2 ). In Fig. 3a , we show the simulated strain profile of a cantilever under pure bending. 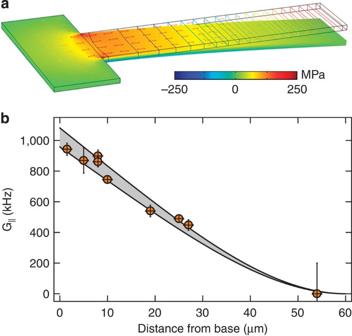Figure 3: Single-spin strain imaging. (a) Stress profile for cantilever used in this experiment at 250 nm of beam deflection using a finite element method simulation. (b) Measured strain coupling (orange circles) as a function of the NV’s distance from the cantilever base for a fixed 250 nm oscillation amplitude. The grey shaded area shows the region of expected strain couplings from theory including uncertainties in NV depth (13 nm) and amplitude of driven motion (10 nm). Vertical error bars correspond to the standard error from fits to the expected control sequence signal. Horizontal error bars correspond to the uncertainty in the NV’s lateral position. Figure 3b shows the measured strain couplings for several NVs along the cantilever for a fixed drive. The data are in good agreement with the theoretical strain profile, shown by the shaded region in Fig. 3b ( Supplementary Note 3 ). Notably, this agreement provides convincing evidence that strain is responsible for the spin evolution. From the data in Fig. 3b , we can extract d ‖ by combining the interferometrically measured amplitude of motion, the NV’s position and orientation in the cantilever, and the expected strain profile of the cantilever ( Supplementary Note 4 ). By measuring several NVs, we average over the variations in NV depth and local strain inhomogeneities, and we find an average value of d ‖ =13.4±0.8 GHz per strain, and hence calibrate our strain sensor. Given our current experimental parameters, we estimate an axial strain sensitivity of approximately 3 × 10 −6 strain Hz −1/2 ( Supplementary Note 5 ). For the cantilevers in this experiment, an NV at the base could then detect ~7 nm of motion in a 1 sec measurement. Figure 3: Single-spin strain imaging. ( a ) Stress profile for cantilever used in this experiment at 250 nm of beam deflection using a finite element method simulation. ( b ) Measured strain coupling (orange circles) as a function of the NV’s distance from the cantilever base for a fixed 250 nm oscillation amplitude. The grey shaded area shows the region of expected strain couplings from theory including uncertainties in NV depth (13 nm) and amplitude of driven motion (10 nm). Vertical error bars correspond to the standard error from fits to the expected control sequence signal. Horizontal error bars correspond to the uncertainty in the NV’s lateral position. Full size image Transverse strain detection We next measured the transverse strain coupling. To do so, we measured NVs oriented perpendicular to the cantilever stress, as shown in Fig. 4a . Although the stress is entirely perpendicular to NVs oriented [ ] and [ ] (shown with red bonds), these NVs will experience non-negligible axial strain in addition to transverse strain because of the Poisson effect [25] . Experimentally, the effects of axial and transverse strains are identified by beatnotes present in the spin evolution. To enhance our sensitivity to these beatnotes, we applied an XY-4 control sequence [26] ( Fig. 4b ) to the NV and decreased B z to 16 G. This sequence increases our sensitivity by extending the coherence time, correcting for first-order timing errors, and increasing the interrogation time. The data and fit to the expected XY-4 signal ( Supplementary Note 6 ) in Fig. 4c give G ⊥ =6.7±0.4 MHz, G ‖ =(2.7±0.5) × 10 2 kHz and a cantilever frequency , in agreement with the cantilever drive frequency of 884.890 kHz. Transforming the cantilever strain tensor into the NV’s coordinate system and using the Poisson ratio of 0.069 for CVD diamond [25] ( Supplementary Note 4 ), we extract d ‖ =13.3±1.1 GHz per strain and d ⊥ =21.5±1.2 GHz per strain. The extracted value of d ‖ is in very good agreement with the extracted value of d ‖ measured for the NVs experiencing predominantly axial strain in Fig. 3 . 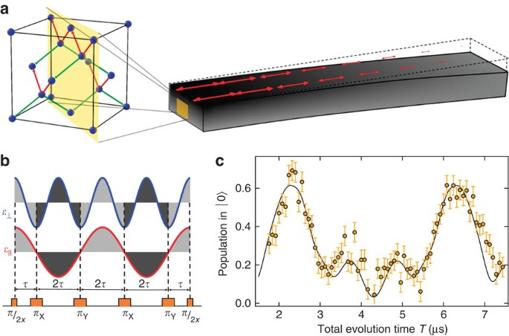Figure 4: Measurement of transverse strain. (a) Stress profile for a cantilever during bending (red arrows). The face of the cantilever (gold square) corresponds to the (110) plane. NVs oriented along [] and [] (red bonds) experience mostly transverse strain, with a small axial strain because of the Poisson effect25. NVs oriented along [111] and [] (green bonds) experience predominantly axial strain (seeSupplementary Information). Measurements of transverse strain are done with NVs oriented [] and []. (b) XY-4 pulse sequence used to measure transverse strain. Transverse strain (in blue) modulates the qubit splitting approximately twice as fast as axial strain (in red). (c) XY-4 spin population (seeSupplementary Information) for an NV (yellow circles) 3 μm from the base with a beam deflection of 675 nm. The expected XY-4 signal for a model considering both axial and transverse strain is shown in black. Error bars correspond to photon counting noise. Figure 4: Measurement of transverse strain. ( a ) Stress profile for a cantilever during bending (red arrows). The face of the cantilever (gold square) corresponds to the (110) plane. NVs oriented along [ ] and [ ] (red bonds) experience mostly transverse strain, with a small axial strain because of the Poisson effect [25] . NVs oriented along [111] and [ ] (green bonds) experience predominantly axial strain (see Supplementary Information ). Measurements of transverse strain are done with NVs oriented [ ] and [ ]. ( b ) XY-4 pulse sequence used to measure transverse strain. Transverse strain (in blue) modulates the qubit splitting approximately twice as fast as axial strain (in red). ( c ) XY-4 spin population (see Supplementary Information ) for an NV (yellow circles) 3 μm from the base with a beam deflection of 675 nm. The expected XY-4 signal for a model considering both axial and transverse strain is shown in black. Error bars correspond to photon counting noise. Full size image The measured strain susceptibility parameters indicate that while the simple model equating strain and electric field accurately predicts the qualitative nature of the NV–strain coupling, it fails to capture the quantitative nature of the strain susceptibility parameters. In particular, this model predicts a value of d ‖ that is approximately 50 times smaller than d ⊥ (ref. 18 ), whereas our measurements show that d ‖ is approximately 1.5 times smaller than d ⊥ . During the preparation of this manuscript, a closely related study [27] reported measurements of d ‖ =5.46±0.31 GHz per strain and d ⊥ =19.63±0.40 GHz per strain using static bending of diamond cantilevers. In comparison with our results, we find good agreement with their value of d ⊥ and find that their value of d ‖ is approximately three times smaller than our measured value. We make several observations in regards to this discrepancy. First, Teissier et al. [27] report large variations (up to one order of magnitude) in the strain susceptibility parameters across NVs. Second, the AC sensing techniques used in our work are inherently more sensitive than the techniques used in ref. 27 , and hence, the amplitude of cantilever bending is significantly smaller here. Large bending amplitudes could lead to deviations from Euler–Bernoulli theory. Furthermore, the resonance phenomenon we utilize provides a well-defined mode shape, whereas static bending may not isolate a single mode. Another study [23] measured shifts of the NV ground-state crystal field splitting under hydrostatic pressure, and their measured value of d ‖ =17.5 GHz per strain is in good agreement with our result. However, no value of d ⊥ was reported. Ab initio calculations from ref. 23 estimate a value of d ‖ =7.44 GHz per strain by considering modifications of the spin–spin coupling because of changes in the NV bond lengths. This value is of the same order of magnitude as our result, indicating that this effect has a significant role in the NV–strain interaction. Looking towards quantum applications [12] , our cantilever’s current zero point motion coupling of g ⊥ =0.04 Hz may be significantly increased by miniaturizing the resonator. For instance, a doubly clamped beam with dimensions of (2 μm, 50 nm, 50 nm) and has a coupling g ⊥ ≈180 Hz. Although having smaller strain couplings than, for example, quantum dot systems where the coupling can be hundreds of kHz (ref. 28 ), the NV centre benefits from its long T 2 coherence times. Assuming T =100 mK, a mechanical Q =10 6 and a T 2 =100 ms, this doubly clamped beam achieves a single spin cooperativity, , where γ = ω m / Q is the damping rate and is the average thermal occupation number of the mechanical mode. We note that although smaller resonators would produce a larger g ⊥ , clamping losses would limit their Q s [29] . At T ≲ 50 K, SCD resonators have demonstrated [11] Q >10 6 . In the devices described here, the Hahn echo T 2 times are roughly 10 μs. Using NVs formed by a nitrogen delta-doping technique [30] and applying higher order dynamical decoupling, longer T 2 times are possible [31] and recently, a T 2 >500 ms has been measured at low temperatures [32] . A cooperativity η >1 enables experiments in the quantum regime that are mediated by a coherent spin–phonon interaction [12] . We note that the strain coupling to the orbital levels of the excited state is significantly higher [4] , [13] , and for the resonator described above, would give a coupling g ⊥ of several MHz, which presents an alternative route to accessing the quantum regime. In conclusion, we have presented a novel hybrid system in which a single NV centre spin is strain-coupled to the mechanical motion of a macroscopic cantilever. We quantitatively measured the NV ground-state spin coupling to axial and transverse strain, and these results will guide theoretical investigations of the strain coupling mechanism. Although our measurements indicate that shear does not couple significantly to the ground-state spin levels of the NV centre, we note that the cantilever-based technique presented here can be extended in future experiments to probe effects of shear on the NV. Furthermore, the coherent strain detection approach we have presented can be extended to other solid-state spin systems, such as SiC colour centres [33] , [34] . With its atomic-scale spatial resolution, NV-based strain sensing could be useful for identifying the poorly understood origins of dissipation in mechanical resonators, such as anchoring losses, which will be instrumental in engineering higher Q resonators [35] . Moreover, our results will provide insight into the role of strain-induced decoherence that could ultimately limit the effectiveness of many NV-based applications [12] , [36] , [37] . Most importantly, we demonstrated that our system provides a feasible route to accessing coherent spin–phonon interactions, with applications ranging from quantum control of a macroscopic resonator to long-range spin–spin interactions. Experimental setup and sample preparation The experimental setup consists of a home-built confocal microscope with an integrated vacuum chamber. The experiments are done at room temperature and high vacuum (~10 −5 Torr) to reduce mechanical dissipation in the resonators. A continuous wave laser at 532 nm is used for optical pumping and readout of the NV spin, and is gated with an acousto-optic modulator (AOM). Photons emitted by the NV into the phonon sideband are collected into a single-mode fibre and directed to a fibre-coupled avalanche photodiode. For strain measurements, the degeneracy of the m s =±1 spin levels is broken by a DC magnetic field supplied by a rare earth magnet. Microwaves used for resonant spin manipulation are delivered to the sample by a wire that sits approximately 30 μm above the sample. Phase control of the microwave pulses is accomplished via IQ modulation. Timing of the pulse sequences is controlled by a Spincore Pulseblaster ESR-Pro 500 MHz card. The cantilevers used in this experiment were fabricated using the techniques described in ref. 10. NVs were formed by 14 N ion implantation with a dosage of 3 × 10 9 ion cm −1/2 at 40 keV and a 0° tilt, which yields an expected depth of 51.5 nm (calculated by Stopping and Range of Ions in Matter (SRIM)). The sample was annealed under high vacuum (~10 −6 Torr) at 800 °C for 3 h. The cantilevers are resonantly driven with a piezoelectric transducer that is clamped to the sample holder and electrically driven with a lock-in amplifier (Zurich Instruments). The cantilevers’ mechanical properties are characterized using standard optical interferometry techniques, as described in ref. 10 . For our experiments, it is very important that we know the amplitude of driven motion of the cantilever. This is calibrated by finding the piezo voltage at which the tip of the cantilever hits the silicon substrate that sits 1 μm below the cantilever. This is measured by an interruption of the Bessel fringes in the interferometric signal. Error analysis Errors in the extracted axial strain coupling parameters and resonator frequencies are given by the standard error in the fit where the couplings and the resonator frequency are the only free parameters. The error in the quoted axial strain susceptibility parameter is given by the standard error in the average value of those parameters as measured by nine NVs. The error in the transverse strain coupling and susceptibility parameter are given by the measurement of a single NV, and the standard error of the fit shown in Fig. 4c . How to cite this article : Ovartchaiyapong, P. et al. Dynamic strain-mediated coupling of a single diamond spin to a mechanical resonator. Nat. Commun. 5:4429 doi: 10.1038/ncomms5429 (2014).